Enantiomeric glycosylated cationic block co-beta-peptides eradicateStaphylococcus aureusbiofilms and antibiotic-tolerant persisters The treatment of bacterial infections is hindered by the presence of biofilms and metabolically inactive persisters. Here, we report the synthesis of an enantiomeric block co-beta-peptide, poly(amido-D-glucose)- block -poly(beta-L-lysine), with high yield and purity by one-shot one-pot anionic-ring opening (co)polymerization. The co-beta-peptide is bactericidal against methicillin-resistant Staphylococcus aureus (MRSA), including replicating, biofilm and persister bacterial cells, and also disperses biofilm biomass. It is active towards community-acquired and hospital-associated MRSA strains which are resistant to multiple drugs including vancomycin and daptomycin. Its antibacterial activity is superior to that of vancomycin in MRSA mouse and human ex vivo skin infection models, with no acute in vivo toxicity in repeated dosing in mice at above therapeutic levels. The copolymer displays bacteria-activated surfactant-like properties, resulting from contact with the bacterial envelope. Our results indicate that this class of non-toxic molecule, effective against different bacterial sub-populations, has promising potential for the treatment of S. aureus infections. Antimicrobial resistance in bacteria is a serious and growing clinical problem, eroding the therapeutic armamentarium and leaving limited treatment options for certain infections. Compounding the difficulty of treating antibiotic-resistant strains is the presence of persisters, subpopulations that are antibiotic-tolerant due to metabolic inactivity [1] , [2] , and the capacity of bacteria to develop biofilms [3] , both of which lead to chronic and recurrent infections [4] , [5] , [6] , [7] . The World Health Organization (WHO) recently published a priority list of bacteria for which new antibiotics are urgently needed [8] . Methicillin-resistant Staphylococcus aureus (MRSA), a WHO high-priority pathogen, is a leading cause of mortality due to antibiotic-resistant infections [9] , [10] . Initially restricted to hospitals and healthcare settings, MRSA is causing an increasing number of infections in the community [11] , [12] . MRSA is associated with poor clinical outcomes [13] : it causes frequent skin and soft tissue infections [14] and can disseminate, resulting in life-threatening bloodstream infections, endocarditis, bone and joint infections, as well as pneumonia [15] , [16] . S. aureus is prone to form biofilms and also exists in the form of metabolically inactive antibiotic-tolerant persister phenotype [3] . Last-resort antibiotics such as vancomycin are largely ineffective against S. aureus persisters and biofilms [17] . New therapeutics are needed to combat the spread of difficult to treat drug-resistant S. aureus infections. Alternative antibacterial agents should have bactericidal activity against replicating cells, persisters, and established biofilms. Cationic alpha-peptides and membrane-active agents have been investigated as alternative antimicrobials to combat biofilms and persisters [18] , [19] , but unselective toxicity is a complicating factor [20] . Amongst the various synthetic polymer families being explored as peptidomimetics [21] , [22] , [23] , [24] , [25] , beta-peptides are promising because they can exhibit biological activity comparable to natural peptides, but have better proteolytic stability [26] , and are usually amphiphilic and non-mutagenic [27] . Beta-peptides have been considered for use in diverse therapeutic applications such as antimicrobial agents [28] , [29] , [30] , vaccine drugs [31] , protein–protein interaction inhibitors [32] , [33] , and drug delivery [34] , [35] . Alpha-peptide antimicrobials are known to form facially amphiphilic (FA) structures that enhance the bactericidal properties but tend to be hemolytic and toxic [36] . Compared to alpha-peptides, beta-peptides have an extra methylene group in the backbone. The hydrophobicity of beta-peptides may be tuned by the structure of the side chains. Further, beta-peptides may be designed to form foldamers exhibiting diverse secondary structures, such as helices and beta-sheets [37] , [38] , [39] and complex tertiary and quaternary structures [40] . Munoz-Guerra and colleagues reported the first research on nylon-3 and analogs, which included the synthesis and helical propensity of these beta-peptides [41] , [42] , [43] . In the development of antimicrobial beta-peptides, previous efforts focus mainly on random co-beta-peptides and optimization of their cationic versus hydrophobic beta-lactam residues to reduce hemolysis whilst maintaining a good bactericidal effect [44] , [45] , [46] , [47] . There is no reported work on glycosylated block co-beta-peptides. Block co-poly(beta-peptides) are interesting as they may show unique combinations of properties displayed by the individual blocks, which are as yet under-exploited for the development of next-generation antibacterials. Also, a strategy for the facile synthesis of block co-beta-peptides has not been previously reported. In this study, we report a simple one-shot one-pot anionic ring opening (co)polymerization (AROP) strategy to synthesize a series of enantiomeric block co-beta-peptides, which cannot be made by sequential copolymerization. Two beta-lactam monomers with contrasting reactivities—a protected d -glucose ( DGu p ) beta-lactam and a protected cationic beta- l -lysine ( BLK p ) beta-lactam—can be block copolymerized in one shot. The resulting optimized block co-beta-peptide, PDGu(7)- block -PBLK(13) , is non-cytotoxic and non-hemolytic in vitro. Further, the block co-beta-peptide has interesting biological properties. Unlike classical antibiotics, PDGu(7)- b -PBLK(13) retains potency against MRSA persister cells and biofilms. It is active against both the community-acquired (CA-) and hospital-associated (HA-) MRSA strains. The block copolymer also effectively removes biofilm biomass but the homocationic beta-peptide ( PBLK(20) ) cannot. The block copolymer is bactericidal against MRSA in various murine models of systemic acute and established infections, and also in an ex vivo human skin infection model, while having no in vivo acute toxicity in murine repeated dosing studies. This study opens up possibilities of treatment for recalcitrant MRSA infections. Synthesis of the (co)polymers via one-shot one-pot AROP The monomers N -Cbz- β -lactam- l -lysine ( BLK p ) and O -Bn- β -lactam- d -glucose ( DGu p ) were synthesized and verified by nuclear magnetic resonance (NMR) spectroscopy (Supplementary Methods, Supplementary Figs. 1 – 3 ). 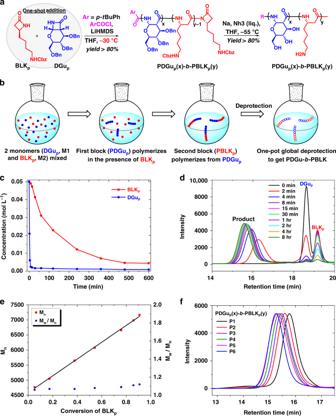Fig. 1 Facile one-shot one-pot synthesis ofPDGu(x)-b-PBLK(y)block copolymer.aSynthetic scheme ofPDGu(x)-b-PBLK(y).bOne-shot addition of both monomers (DGupandBLKp) leads to block copolymerization when the monomers have contrasting reactivities.c–eKinetic studies andfGPC measurements verify the well-controlled single chain block architecture ofPDGup(x)-b-PBLKp(y).cRemaining monomer concentration vs time.dGPC curves of partially polymerized products at selected quenching times.eMolecular weight (Mn) and molecular weight distribution (Đ) as a function of conversion ofBLKp.fGPC of protected-(co)polymers The copolymer synthetic strategy relies on the observation that the homopolymerization of N -Cbz- β -lactam- l -lysine monomer ( BLK p ) is much slower than the homopolymerization of O -Bn- β -lactam- d -glucose monomer ( DGu p ) (Supplementary Table 1 ). When DGu p and BLK p monomers (10:10, mole/mole) were mixed together in tetrahydrofuran, DGu p was totally consumed in 8 min while the BLK p monomer required 8 h for complete reaction (Fig. 1a–c , Supplementary Figs. 4 , 5 ). The molecular weight of the product increased linearly over an 8-h period during which DGu p disappeared rapidly in the first few minutes, while BLK p was consumed gradually over the next few hours (Fig. 1d ). A plot of molecular weight ( M n ) versus BLK p conversion (Fig. 1e ) shows a linear relationship and the Đ values of the products remain small (1.06–1.12). These results are consistent with the growth of a single copolymer chain through rapid consumption of DGu p followed by slower but contiguous incorporation of BLK p , and thus provide evidence for a ‘block-like’ structure of the resulting copolymer. A series of poly(Bn-amido- d -glucose)- block -poly(Cbz-beta- l -lysine) ( PDGu p (x)- b -PBLK p (y) ) block copolymers, with varying ratios of x to y but constant target total degree of polymerization of 20, i.e. ( x + y ) = 20, was synthesized (Fig. 1a , Supplementary Fig. 6 ). The molecular weights are close to the design values based on gel permeation chromatography (GPC) relative to polystyrene standards, confirming that the AROP process is well-controlled (Fig. 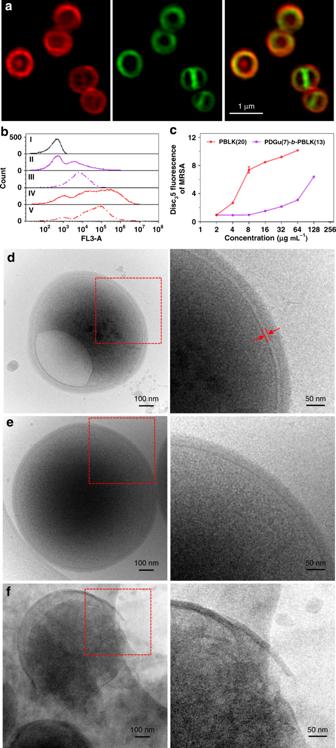Fig. 2 PDGu(7)-b-PBLK(13)targets bacterial cell envelope. It accumulates in MRSA USA300 cell envelope, mildly (at MIC) permeabilizing the membrane but significantly weakening cell wall/membrane attachment.aConfocal microscopy images of copolymer-treated MRSA USA300. From left to right: rhodamine-labeled copolymer channel, FM1-43-labeled bacteria membrane channel, superimposed images from both channels, respectively.bFlow cytometry study of propidium iodide-stained MRSA USA300. From top to bottom: live bacteria control, bacteria treated with 1× MICPDGu(7)-b-PBLK(13), 4× MICPDGu(7)-b-PBLK(13), 1× MICPBLK(20), and 4× MICPBLK(20).cDiSC35 membrane depolarization assay. Data are presented as mean ± standard deviation.d–fCryo-TEM image of polymer treated MRSA USA300.dPDGu(7)-b-PBLK(13)treated bacteria with enlarged periplasmic space and vacuole structure formation;euntreated control;fPBLK(20)-treated bacteria with cell lysis 1f , Supplementary Table 2 ). Fig. 1 Facile one-shot one-pot synthesis of PDGu(x)- b -PBLK(y) block copolymer. a Synthetic scheme of PDGu(x)- b -PBLK(y) . b One-shot addition of both monomers ( DGu p and BLK p ) leads to block copolymerization when the monomers have contrasting reactivities. c – e Kinetic studies and f GPC measurements verify the well-controlled single chain block architecture of PDGu p (x)- b -PBLK p (y) . c Remaining monomer concentration vs time. d GPC curves of partially polymerized products at selected quenching times. e Molecular weight (M n ) and molecular weight distribution ( Đ ) as a function of conversion of BLK p . f GPC of protected-(co)polymers Full size image After one-step deprotection, the final products PDGu(x)- b -PBLK(y) were obtained with overall yields greater than 65% (Supplementary Fig. 7 ). NMR spectroscopy measurements of PDGu(x)- b -PBLK(y) show two sets of signals belonging to PDGu and PBLK , respectively, corroborating their block rather than random structures (Supplementary Figs. 8 – 22 ). NMR spectra also show that the ratios of DGu to BLK in PDGu(x)- b -PBLK(y) after purification deviate slightly from the stoichiometric ratios of added monomers. For example, the actual composition of DGu and BLK in PDGu(10)- b -PBLK(10) is PDGu(7)- b -PBLK(13) ; the PBLK block is 66 mol% versus the design value of 50 mol%. This trend is repeatable and can be seen in other compositions (Table 1 ). The molecular weights (M n ) of the homocationic PBLK(20) , homosugar PDGu(20) , and copolymer PDGu(7)- b -PBLK(13) were, respectively, 3012 Da, 3159 Da, and 3391 Da, as measured by the Matrix Assisted Laser Desorption/Ionization-Time of Flight (MALDI-TOF) mass spectroscopy (Supplementary Fig. 23 ). Table 1 Design and actual ratios of DGu to BLK before and after deprotection Full size table When we attempted the synthesis of PDGu p (10) - b - PBLK p (10) by the sequential addition of DGu p (M1) followed by BLK p (M2) at −30 °C (Supplementary Fig. 24a ), the amount of isolated undesired homopolymer PDGu p after the reaction could be more than 50% of the yield (based on DGu p ). This sequential copolymerization of higher reactivity DGu p followed by lower reactivity BLK p could be finished rapidly in <1 h, but achieved only low purity block copolymer with substantial PDGu p homopolymer. We expected that by reversing the order of addition of monomers, i.e. first BLK p and then DGu p (Supplementary Fig. 24b ), in which the first block ( PBLK p ) has a lower reactivity and also a higher transfer rate to DGu p , the block copolymerization would successfully occur. However, the first step requires up to 8 h to reach ~90% conversion (based on BLK p ). In addition, the final mixture was very viscous and contained a large proportion of pre-mature terminated PBLK p . Regardless of the sequence of monomer addition, sequential copolymerization cannot successfully synthesize cationic glycosylated block copoly(beta-peptide) with good yield and purity. Unexpectedly, with one-shot AROP with simultaneous feed of the two beta-lactams, we could achieve successful synthesis of the block copolymers PDGu p - b -PBLK p . PDGu(7)- b -PBLK(13) is antibacterial and non-cytotoxic The PDGu(x)- b -PBLK(y) series was tested against a panel of Gram-positive bacteria. The homopolymer PBLK(20) was active against most tested bacteria, but was unselective and cytotoxic to eukaryotic cells and also hemolytic (Table 2 , Supplementary Figs. 25 and 26 ). The block copolymerization process decreased cytotoxicity while maintaining potency against S. aureus . The copolymer PDGu(7)- b -PBLK(13) shows the most balanced profile, combining potency against S. aureus with good selectivity index (>25) and no hemolysis (HC 10 > 20,000 µg mL −1 ) (Table 2 , Supplementary Figs. 25 and 26 ). The copolymer shows good activity against USA300 (Table 2 ), the predominant CA-MRSA [11] . 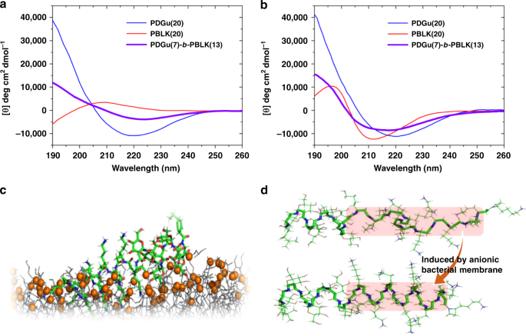Fig. 3 Bacterial-induced secondary structure transition ofPDGu(7)-b-PBLK(13).a,bMolar ellipticity [θ] CD spectra ofPDGu(20)(blue),PBLK(20)(red), andPDGu(7)-b-PBLK(13)(purple) in DI (a) and in the presence of anionic POPG liposomes (b).cA snapshot of computer simulation ofPDGu(7)-b-PBLK(13)binding to anionic bacterial membrane. The membrane model is colored as gray lines with the head groups of the lipid molecules shown as orange spheres.PDGu(7)-b-PBLK(13)is shown as a stick model, its carbon, oxygen, nitrogen, and hydrogen atoms are colored as green, red, blue, and white, respectively.dComputer simulation of transition from helix–coil in solution to helix–helix induced by anionic membrane Further profiling demonstrated that the copolymer is also potent against other MRSA strains from major lineages of global epidemiology [48] , including (HA-)MRSA strains resistant to multiple conventional antibiotics (including vancomycin, daptomycin) (Table 3 ). Kill-kinetics experiments revealed that PDGu(7)- b -PBLK(13) killed replicating MRSA faster than vancomycin (Supplementary Fig. 27 ). The selection of escape mutants to PDGu(7)- b -PBLK(13) at 10× its minimum inhibitory concentration (MIC) was unsuccessful, showing that the propensity for emergence of resistance is extremely low (frequency below 3 × 10 −10 , which is much lower than reported values for antibiotics [49] , [50] ). We then tried to select mutants by the continued pressure of sub-inhibitory concentrations of the block copolymer for up to 14 days (as described previously [51] ). This approach also did not select for copolymer-resistant MRSA colonies. As a control, escape mutants resistant to the antibiotic ciprofloxacin were easily selected (Supplementary Fig. 28 ). Table 2 Antimicrobial and hemolytic activity and biocompatibility of (co)polymers Full size table Table 3 Antimicrobial activity against multi-drug-resistant clinically isolated MRSA Full size table PDGu(7)- b -PBLK(13) targets the bacterial envelope The structure of the cationic block co-beta-peptide suggests a possible mechanism of action involving membrane interaction. Confocal microscopy of fluorescently labeled bacterial cells showed that the rhodamine-labeled PDGu(7)- b -PBLK(13) accumulated preferentially in the bacteria envelope (i.e. cell wall and cell membrane) (Fig. 2a , Supplementary Fig. 29 ). Membrane damage was confirmed using propidium iodide (PI) as a marker of plasma membrane integrity (Fig. 2b ). Results showed that both the block copolymer and cationic homopolymer are membrane active, but the copolymer induces less PI staining, suggesting that it is less membrane-lytic (Fig. 2b ). DiSC 3 5 dye assay, which probes plasma membrane potential changes, corroborated the finding that PDGu(7)- b -PBLK(13) mildly depolarized the bacterial plasma membrane, unlike the homocationic PBLK(20) that had a more pronounced effect (Fig. 2c ). Together, the PI staining and DiSC 3 5 assay results indicate that the copolymer disturbs the bacterial membrane without causing severe leakage. Fig. 2 PDGu(7)- b -PBLK(13) targets bacterial cell envelope. It accumulates in MRSA USA300 cell envelope, mildly (at MIC) permeabilizing the membrane but significantly weakening cell wall/membrane attachment. a Confocal microscopy images of copolymer-treated MRSA USA300. From left to right: rhodamine-labeled copolymer channel, FM1-43-labeled bacteria membrane channel, superimposed images from both channels, respectively. b Flow cytometry study of propidium iodide-stained MRSA USA300. From top to bottom: live bacteria control, bacteria treated with 1× MIC PDGu(7)- b -PBLK(13) , 4× MIC PDGu(7)- b -PBLK(13) , 1× MIC PBLK(20) , and 4× MIC PBLK(20) . c DiSC 3 5 membrane depolarization assay. Data are presented as mean ± standard deviation. d–f Cryo-TEM image of polymer treated MRSA USA300. d PDGu(7)- b -PBLK(13) treated bacteria with enlarged periplasmic space and vacuole structure formation; e untreated control; f PBLK(20) -treated bacteria with cell lysis Full size image The effect of PDGu(7)- b -PBLK(13) on the morphology of S. aureus was also visualized by cryo-transmission electron microscopy (cryo-TEM), which revealed a much larger periplasmic space gap (of about 7–8 nm, Fig. 2d ; indicated by red arrows), together with bleb and vacuole formation (Fig. 2d , Supplementary Fig. 30 ). In contrast, periplasmic gap widening, blebs, and vacuoles were not observed in untreated bacteria (Fig. 2e , Supplementary Fig. 31 ). Treatment with PBLK(20) led to significant bacterial envelope deformation, cell leakage, and lysis (Fig. 2f , Supplementary Fig. 32 ). The copolymer with its hydrophilic sugar block aggregates at the membrane interface, leading to the observed larger periplasmic gap. Circular dichroism (CD) spectropolarimetry showed that in free solution, the block co-beta-peptide likely adopts a helix–coil conformation attributed respectively to the sugar [52] and cationic [53] blocks (Fig. 3a ). However, in the presence of model vesicles containing anionic bacterial lipids, CD spectrum shows that the cationic block of the copolymer, like the cationic homopolymer ( PBLK(20) ), undergoes a transition to likely a left-handed helix structure [54] (Fig. 3b , Supplementary Fig. 33a–f ). Computer simulation shows that the binding of PDGu(7)- b -PBLK(13) to bacterial membrane is provided mainly by the PBLK block while the PDGu block protrudes into the water–membrane interface because of its weaker binding to the membrane and its strong hydrophilicity (Fig. 3c , Supplementary Fig. 34 ). In free solution, electrostatic repulsion between the lysine side chains of the cationic block causes the cationic block to exist as a random coil conformation (Supplementary Fig. 34a–d ). At the anionic bacterial lipid surface, the positive charges in the PBLK block of the copolymer are neutralized by anionic bacterial lipids so that the lysine side chain charge–charge repulsion causing the distortion of the helical conformation of the copolymer PBLK block is substantially reduced and the copolymer transitions from a helix–coil structure to a helix–helix structure (Fig. 3d , Supplementary Fig. 34e–g ). The resulting helix–helix structure of the sugar-cationic block copolymer binds to the anionic bacterial membrane (Supplementary Fig. 34h–k ). It is known that beta peptides containing cyclic beta-amino acids adopt different helical structures to those containing non-cyclic amino acids [39] . From the CD data, we see that the (cyclic) PDGu spectrum exhibited a minimum at 220 nm while the (non-cyclic) PBLK spectrum exhibited a minimum at 213 nm (Fig. 3b ). Our computer simulation corroborated that the PDGu and PBLK blocks adopt different helical conformations, with 3.5 residues/turn and 3 residues/turn, respectively (Supplementary Fig. 34j , Supplementary Note). (In the presence of zwitterionic lipids (model vesicles representative of mammalian membrane), the copolymer retained its helix–coil conformation (Supplementary Fig. 33c )). Fig. 3 Bacterial-induced secondary structure transition of PDGu(7)- b -PBLK(13) . a , b Molar ellipticity [ θ ] CD spectra of PDGu(20) (blue), PBLK(20) (red), and PDGu(7)- b -PBLK(13) (purple) in DI ( a ) and in the presence of anionic POPG liposomes ( b ). c A snapshot of computer simulation of PDGu(7)- b -PBLK(13) binding to anionic bacterial membrane. The membrane model is colored as gray lines with the head groups of the lipid molecules shown as orange spheres. PDGu(7)- b -PBLK(13) is shown as a stick model, its carbon, oxygen, nitrogen, and hydrogen atoms are colored as green, red, blue, and white, respectively. d Computer simulation of transition from helix–coil in solution to helix–helix induced by anionic membrane Full size image The accumulation of the block co-beta-peptide at the outer leaflet of the cytoplasmic membrane causes the increased periplasmic space visible in the cryo-TEM (Fig. 2d ), which led to detachment of the cell wall from the cytoplasmic membrane and a weakened membrane–cell wall interface. The copolymer also aggregates inside the cell wall leading to defects in the cell wall function (Fig. 2a, d ). The blebs observed with copolymer treatment using cryo-TEM (Supplementary Fig. 30 ) may be formed by membrane-bound cytoplasm herniating through cell wall defects as intracellular water expands during the freezing process of the cryo-TEM preparation [55] , [56] . The vacuoles observed (Supplementary Fig. 30 ) may be ice pockets formed during the cryo-TEM process as water migrates to the polymer-rich periplasmic space since the cytoplasmic membrane is detached from the cell wall. Taken together, the copolymer disturbs the cell envelope which includes the membrane, the membrane–cell wall interface, and also the cell wall. PDGu(7)- b -PBLK(13) eradicates persister bacteria and biofilms Classical antibiotics are usually significantly less potent against persisters/non-replicating bacteria [1] , [2] , [6] , [7] . Since PDGu(7)- b -PBLK(13) kills S. aureus by surface contact-induced membrane/envelope damage, we hypothesized that the block copolymer may retain potency against persisters and S. aureus biofilms [18] . Nutrient-starved persisters were generated by passaging S. aureus in PBS medium, a condition under which the bacteria can survive for extended periods of time without replicating. Consistent with published literature [1] , non-replicating S. aureus was phenotypically resistant to antibiotics from various categories (including vancomycin, oxacillin, rifampicin, etc.) up to a dose 100× MIC (Fig. 4a ). Conversely, PDGu(7)- b -PBLK(13) was highly potent against non-replicating starved persister S. aureus at a concentration as low as twofold its MIC (Fig. 4b ). Furthermore, PDGu(7)- b -PBLK(13) effectively eradicated antibiotic-induced persisters that escaped killing by 10× MIC gentamicin and ciprofloxacin treatment (Fig. 4c, d ). PDGu(7)- b -PBLK(13) was also effective at dispersing preformed MRSA biofilms, achieving a reduction of more than 99.9% of the biofilm bacteria, greatly outperforming vancomycin, which had an insignificant effect on biofilm bacteria (Fig. 4e ). Fig. 4 PDGu(7)- b -PBLK(13) is bactericidal toward MRSA USA300 persisters and biofilms in vitro. a Kill-kinetics of various antibiotics at 100× MIC; and b PDGu(7)- b -PBLK(13) against non-replicating MRSA USA300. c , d Kill-kinetics of PDGu(7)- b -PBLK(13) at 4× MIC against persisters generated by 10× MIC gentamicin ( c ) and ciprofloxacin ( d ) treatment. e Activity of PDGu(7)- b -PBLK(13) and PBLK(20) on established MRSA biofilms using the MBEC™ Assay. Data are presented as mean ± standard deviation. f FESEM image of MBEC™ microtiter plate pegs: (left) control peg without treatment and (right) peg treated with PDGu(7)- b -PBLK(13) . g , h Confocal microscopy images of PDGu(7)- b -PBLK(13) ( g ) and PBLK(20) ( h ) treated MRSA biofilm at t = 0 min, 30 min, and 3 h. Biofilms were stained with Live/Dead BacLight™ kit Full size image In addition to killing bacteria in biofilm, the block copolymer effectively dispersed the biofilm itself (as shown by confocal microscopy and FESEM) and the dispersed bacteria were shown to be dead (Fig. 4f, g , Supplementary Fig. 35a, b ). The homocationic PBLK(20) kills biofilm bacteria but does not disperse them (Fig. 4e, h , Supplementary Fig. 35c ). Copolymer aggregation at the cell wall accounts for its ability to detach bacteria from biofilm biomass since the sugar block would form a non-fouling coating around the bacteria. (CA-)MRSA USA300 maintained in a broth medium supplemented with glucose typically forms biofilm involving cell-wall anchored protein (fibronectin-binding proteins) [57] , whilst many (HA-)MRSA [58] , [59] and Staphylococcus epidermidis [60] , [61] strains form biofilms involving the polysaccharide intercellular adhesin encoded by the ica locus [62] . To determine if the block copolymer is active against other types of biofilms, biofilms formed by various HA-MRSA and methicillin-resistant S. epidermidis (MRSE) strains under conditions promoting the ica locus expression [63] were treated with the copolymer. Our copolymer PDGu(7)- b -PBLK(13) was more active than vancomycin in eradicating the biofilms of HA-MRSA and MRSE strains (Fig. 5 ). Hence, our copolymer is effective not only against MRSA biofilms involving fibronectin-binding protein, but also against other major types of biofilm formed by HA-MRSA and MRSE. Fig. 5 PDGu(7)- b -PBLK(13) eradicates biofilms of HA-MRSA and MRSE strains. It shows dose-dependent eradication of biofilm bacteria under conditions that promote polysaccharide intercellular adhesion; y -axis: biofilm bacteria (CFU mm −2 peg) formed by different HA-MRSA strains ( a ATCC BAA38, b ATCC BAA39, c ATCC BAA40, d ATCC BAA44) and MRSE strains ( e ATCC 35984, f ATCC 700563). (Vancomycin is used as antibiotic control.) Data are presented as mean ± standard deviation Full size image Copolymer is efficacious in murine and ex vivo human skin models Before in vivo efficacy testing, acute toxicity of the block copolymer was evaluated in mice. Intravenous injection of PDGu(7)- b -PBLK(13) at a cumulative dose of 70 mg kg −1 (10 mg kg −1 per day × 7 days) was well tolerated in all mice, with no death observed up to 7 days post-injection (Fig. 6a ). PDGu(7)- b -PBLK(13) induced no liver and kidney toxicity, confirming its low in vivo acute toxicity (Fig. 6b , Supplementary Fig. 36 , Supplementary Table 3 ). Fig. 6 PDGu(7)- b -PBLK(13) is efficacious in vivo against MRSA USA300 with no toxicity. a , b In vivo repetitive toxicity of daily 10 mg kg −1 i.v. injection of PDGu(7)- b -PBLK(13) for 7 consecutive days. a Mice weight (left y -axis) and cumulative dosage (right y -axis) over 14 days. b ALT and AST biomarker changes at t = 0 and 7 days. Data are presented as mean ± standard deviation. c Survival% and d bacteria log reduction in liver in a systemic infection model. Vehicle alone (–), PDGu(7)- b -PBLK(13) , or vancomycin control at 5 mg kg −1 were applied at a single dose, 2-h post infection. e In vivo antimicrobial activity of PDGu(7)- b -PBLK(13) against MRSA USA300 in a deep-seated neutropenic thigh infection model. First treatment was applied 24-h post infection at 20 mg kg −1 , with a second dose at 20 mg kg −1 applied 3 h later. f In vivo antimicrobial activity of PDGu(7)- b -PBLK(13) against MRSA USA300 in an established murine excision wound model. Vehicle alone (–), PDGu(7)- b -PBLK(13) , or vancomycin control at the same dosing (i.e. 2.5 mg kg −1 ) were applied six times over 2 days, starting 72-h post infection. g Ex vivo antimicrobial activity of PDGu(7)- b -PBLK(13) against MRSA USA300 in an established wounded human skin model. Vehicle alone (–), PDGu(7)- b -PBLK(13) , or vancomycin control at 100 µg were applied three times with 3-h interval between treatments, starting 48 h post infection; ** p ≤ 0.01, *** p ≤ 0.001, **** p ≤ 0.0001 by one-way ANOVA followed by Dunnett test Full size image The in vivo efficacy of PDGu(7)- b -PBLK(13) was then evaluated in a mouse model of acute systemic infection. Mice were infected with MRSA USA300 at a lethal dose (100% death within 24 h in untreated controls). At 2 h post infection, a single 5 mg kg −1 dose of intraperitoneally (i.p.) injected copolymer resulted in 100% rescue of the mice (6/6 mice) and significantly reduced bacterial loads in major organs (Fig. 6c, d , Supplementary Fig. 37 ). In contrast, vancomycin treatment at the same dosage achieved only 67% survival (4/6 mice). We further evaluated the efficacy of the copolymer against persisters/biofilm with a deep-seated thigh infection model in neutropenic mice known to be particularly resistant to antibiotic treatment [18] , [64] . In this model, the copolymer achieved a 93.7% (1.2 log 10 ) reduction in bacteria load, whereas vancomycin was ineffective (Fig. 6e ). We also evaluated the efficacy of the co-beta-peptide against biofilm bacteria in a murine excision wound model. A biofilm was established in the wound with a 72-h infection period, by which time the bacteria have developed stable biofilms [65] , [66] . After the 72-h infection, copolymer treatment was given and achieved 99.87% (2.9 log 10 ) reduction in bacterial load, which was significantly better than vancomycin (83.8%, i.e. 0.8 log 10 , reduction) (Fig. 6f ), showing that the block copolymer has high activity even against an established S. aureus infection known to be recalcitrant to antibiotic treatment. In addition to the murine models, we also demonstrated the efficacy of the copolymer with an ex vivo human skin model with severely established (48 h) infection (Fig. 6g ). The copolymer treatment achieved 99.998% (4.6 log 10 ) reduction of bacterial burden in contrast to the 97.3% (1.6 log 10 ) reduction of vancomycin treatment. Copolymer treated ex vivo human wound sites were also clear of pus/debris corroborating its anti-fouling/biofilm dispersal properties (Supplementary Fig. 38 ). Eradication of persisters and biofilms remains one of the biggest challenges in antibacterial drug discovery. Antibiotic-tolerant bacteria are associated with longer treatment time and relapse of infection. Because most antibiotics target macromolecular machinery only essential for active replication, they are significantly less potent against non-replicating persisters or established biofilms. PDGu(7)- b -PBLK(13) kills non-replicating, antibiotic-tolerant persisters, and biofilm-associated MRSA, both in vitro and in vivo. We show that it can eradicate the clinically relevant CA-MRSA (USA 300). We also showed that our copolymer is just as effective against HA-MRSA strains with resistance to multiple conventional antibiotics (Table 3 , Fig. 5 ). Multi-drug-resistant (MDR) HA-MRSA bacteria cause the majority of nosocomial bacteremia/septicemia and device-related infections involving biofilm formation. The ability of our co-beta-peptide to kill all the sub-populations (planktonic, persister and biofilm states) of MRSA bacteria is attributable to its mechanism(s) of kill—membrane disruption and interface weakening effects which are not related to metabolism. The reduced tendency of the block copolymer to bind mammalian membranes is linked to their less negatively charged surface [36] , [67] . This co-beta-peptide shows eradication of persister and biofilm MRSA and has ultra-low toxicity, both of which were shown using in vivo murine models. Further, it also shows eradication of an established infection with an ex vivo human skin model. Upon surface-contact with bacterial membrane, the cationic block undergoes transition from a random coil in free solution to a helix. The block copolymer possesses a unique bacteria-triggered surfactant effect that contributes to biofilm dispersal—the cationic block adsorbs onto the negatively charged bacterial envelope while the hydrophilic sugar block has a strong tendency to promote dissolution, resulting in a “surfactant-like” solvation of bacteria from biofilm. The block copolymer forms an anti-fouling PDGu layer around the bacteria. Conversely, the homocationic PBLK(20) led to pore formation (Fig. 2b, c, f ), like other AMPs [36] , but without promoting biofilm detachment (Fig. 4h ); this is probably linked to the inability of the homocationic polymer to form an anti-fouling layer around the bacteria. The amine group of the cationic block dominates the interactive topology with erythrocytes but its hydrophilicity minimizes hemolysis. Further, the neutral sugar block also increases the hydrophilicity of the block copolymer. Other antimicrobial peptides and biosurfactants (such as surfactin, rhamnolipid, or phenol-soluble modulins) are intrinsically amphiphilic with exposed hydrophobic domains in free solution and are typically hemolytic since their freely exposed hydrophobic moieties would interact with erythrocytes [68] . Biofilm eradication using conventional antibiotics is typically challenging [69] , [70] . The limited efficacy of vancomycin against biofilms is not an exception; many other antibiotics that are commonly used for MRSA infection have significantly reduced efficacy against biofilm bacteria [71] . 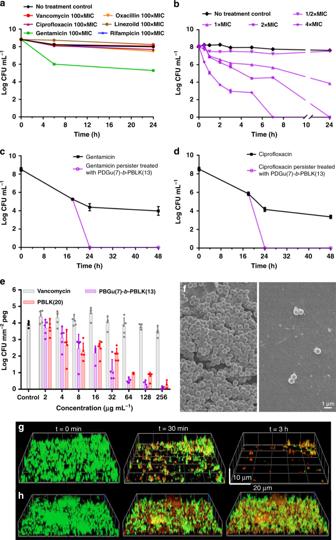Fig. 4 PDGu(7)-b-PBLK(13)is bactericidal toward MRSA USA300 persisters and biofilms in vitro.aKill-kinetics of various antibiotics at 100× MIC; andb PDGu(7)-b-PBLK(13)against non-replicating MRSA USA300.c,dKill-kinetics ofPDGu(7)-b-PBLK(13)at 4× MIC against persisters generated by 10× MIC gentamicin (c) and ciprofloxacin (d) treatment.eActivity ofPDGu(7)-b-PBLK(13)andPBLK(20)on established MRSA biofilms using the MBEC™ Assay. Data are presented as mean ± standard deviation.fFESEM image of MBEC™ microtiter plate pegs: (left) control peg without treatment and (right) peg treated withPDGu(7)-b-PBLK(13).g,hConfocal microscopy images ofPDGu(7)-b-PBLK(13)(g) andPBLK(20)(h) treated MRSA biofilm att= 0 min, 30 min, and 3 h. Biofilms were stained with Live/Dead BacLight™ kit Besides antibiotics, our copolymer outperforms many cationic antimicrobial peptides and conventional antiseptic therapeutics in established wound infections that have been previously reported [19] , [72] , not to mention its superior safety profile that makes it suitable for translation into clinics. The copolymer eradicates biofilm MRSA and also disperses the biomass. Since the block copolymer forms an anti-fouling PDGu coating around the bacterial cell envelope, the adhesion of the bacteria to extracellular polymeric substances (EPSs) and to substrates is reduced, explaining the strong dispersing effect of PDGu(7)- b -PBLK(13) on biofilms (Fig. 4e ). The coated bacteria can effectively detach due to reduced surface hydrophobicity and interaction with biofilm matrix, leading to biofilm dispersal [73] , [74] , [75] . Moreover, the copolymer biofilm eradication effect is observed in the major types of biofilms formed by different MRSA (and MRSE) strains under various conditions, which include the types involving fibronectin binding protein as well as polysaccharide intercellular adhesin. This is clinically significant since MRSA is a common pathogen that forms biofilms during infection, as well as on medical devices [15] , [76] . The block co-beta-peptide ( PDGu(7)- b -PBLK(13) ) demonstrates excellent bactericidal efficacy against all MRSA sub-populations, i.e. replicating, biofilm-associated, and antibiotic-induced persister bacteria. It is active against CA-MRSA (USA300) and numerous other MDR HA-MRSA. The cationic block co-beta-peptide undergoes a bacterial-membrane-triggered conformation change from a random coil to likely a helix. Its antibacterial activity in established MRSA murine infection models is superior to that of vancomycin, and it exhibits no acute in vivo toxicity in repeated dosing studies at levels above those required for therapeutic efficacy. Further, the copolymer effectively eradicates established MRSA infections in an ex vivo human skin model. It also kills biofilm bacteria while effectively dispersing the biofilm mass of CA-MRSA; it also shows efficacy against the major types of biofilms formed by HA-MRSA. It acts as a bacteria-triggered surfactant leading to biofilm dispersal. As resistance toward all classes of antibiotics rapidly evolves and spreads [77] , the outstanding efficacy of PDGu(7)- b -PBLK(13) against S. aureus persisters and biofilms, as well as its excellent safety window, makes this block co-beta-peptide a valuable candidate to treat MRSA infections. General procedure for the polymerization of β-lactams In a nitrogen-purged glovebox, a mixture of two β -lactams ( BLK p and DGu p ) dissolved in tetrahydrofuran with a defined molar ratio was placed into a Schlenk tube equipped with a magnetic stirrer (Fig. 1a). Then, 4- t -butylbenzoyl chloride (tBuBzCl, 5 mol% with respect to the total amount of β -lactam) was added. The Schlenk tube was sealed, removed from the glove box, and cooled to −30 °C under argon atmosphere. To the stirring reaction solution was then slowly added a premade stock solution of lithium bis(trimethylsilyl)amide (LiHMDS, 12.5 mol% with respect to the total amount of β -lactam). The resulting mixture was stirred at −30 °C for about 8 h until the reaction was finished (monitored by TLC) and was then quenched with methanol. After completion, a white solid was precipitated by adding hexane (40 mL). The mixture was centrifuged and the supernatant solution was decanted. After two more repetitions of the precipitation/centrifugation procedure, the white pellet was dried overnight under a nitrogen stream to yield the protected product PDGu p (x)- b -PBLK p (y) as a white powder. General procedure for the debenzylation of PDGu p (10)- b -PBLK p (10) Polymer PDGu p (10)- b -PBLK p (10) (145 mg) and 54 mg (0.48 mmol, ~1.2 equiv. to monomers) of potassium tert -butoxide (KO t -Bu) were dissolved in 5.0 mL of tetrahydrofuran. The polymer solution was added dropwise to a rapidly stirred solution of sodium (160 mg, 7.0 mmol) in liquid ammonia (15 mL) at −78 °C under nitrogen. The reaction mixture was warmed to −55 °C and maintained at this temperature for about 2 h, after which a saturated aqueous solution of ammonium chloride (NH 4 Cl, 10 mL) was added to quench the reaction. The solution was warmed to room temperature in a water bath to evaporate the ammonia. The resulting clear solution was filtered, washed with DI water, and dialyzed with 1000 MWCO tubing for 36 h with ten water changes. After lyophilization, PDGu(7)- b -PBLK(13) was obtained as an amorphous white solid. Copolymers ( PDGu p (x)- b -PBLK p (y) ) with other design block lengths ( x , y ) were synthesized by a similar procedure. Reaction kinetics studies High-performance liquid chromatography (HPLC) was employed to determine β -lactam consumption. For these measurements, a series of reactions was performed with identical conditions (temperature: −30 °C, initial concentration: [ DGu p ] = 0.05 M, [ BLK p ] = 0.05 M, activator [ArCOCl] = 0.005 M, inititator [LiHMDS] = 0.0125 M) but quenched at different times. After purification by flash column chromatography, concentrated reaction mixtures were mixed with a certain amount of paraben (internal standard) and diluted with acetonitrile to the same volume. Aliquots of these solutions were transferred to vials and injected into a Shimadzu LC-20AD HPLC workstation equipped with an IB column. Monomer concentration was calculated from the peak area ratio relative to a known amount of internal standard. GPC curves were determined versus polystyrene standards using dimethylformamide (1 mg mL −1 LiBr) as the eluent at a flow rate of 1.0 mL min −1 through two Styragel columns (HR5 and HR5E, 7.8 × 300 mm) in series at 40 °C with a refractive index detector. Bacterial strains All bacteria strains of Table 2 , Strains #14–17 of Table 3 , and all bacteria strains of Fig. 5 were purchased from ATCC. Vancomycin-resistant S. aureus (Strains #1–7 of Table 3 ) were kindly provided by Prof. Barry N. Kreiswirth and Dr. José R. Mediavilla from the Center for Discovery and Innovation, Hackensack Meridian Health (USA). Daptomycin non-susceptible vancomycin-intermediate MRSA (Strains #8 and 9 of Table 3 ) were kindly provided by BEIresources.org. Strain #10 of Table 3 was kindly provided by Dr. Adriana Rosato from the Houston Methodist Research Institute (USA). Strains #11–13 of Table 3 were kindly provided by Tan Tock Seng Hospital (TTSH, Singapore). Multilocus sequence typing (MLST) characterization for the three VISA strains from local hospital (Strains #11–13 of Table 3 ) were conducted. Overnight culture from single colony was washed with 10 mM Tris buffer, resuspended in 800 µL of lysis buffer containing 5 mg mL −1 lysozyme, 10 mM EDTA, and 10 mM Tris. After 1 h incubation at 37 °C with shaking, the suspension was heated to 95 °C for 10 min and subsequently transferred to ice. 1 mL of ice-cold phenol/chloroform/isoamyl alcohol (25:24:1) was added and mixed thoroughly by inverting the tubes five times, followed by incubation for 5 min on ice. After centrifugation at 20,000× g for 20 min, the aqueous layer was transferred to a fresh tube and DNA was precipitated by adding 1 mL of ice-cold ethanol, followed by incubation for 15 min on ice. The DNA pellet was collected by centrifugation and washed once with ice-cold 70% ethanol, and resuspended in 50 µL of water. The extracted DNA were amplified by PCR using Novagen KOD Hot Start DNA Polymerase, and the amplified products were sequenced by Sanger sequencing. The obtained sequence was submitted to MLST database ( http://www.mlst.net/ ) to obtain the sequence type (ST). MIC determination Bacteria in logarithmic phase of growth were diluted to 1 × 10 6 colony-forming units (CFU) per milliliter in Mueller Hinton Broth (MHB, Difco ® ). Polymers were dissolved at 10.24 mg mL −1 in deionized water and diluted to desired concentration in MHB using twofold serial dilution in a 96-well plate (Nunc TM ). A total of 50 µL of bacteria in MHB suspension were added to 50 µL of polymer to achieve a final volume of 100 µL per well. The plate was incubated aerobically at 37 °C for 18 h, and the optical density of each well was measured at a wavelength of 600 nm (TECAN, infinite F200). MIC 90 is defined as the lowest concentration that exhibited more than 90% inhibition of the bacteria growth. All tests were performed three times independently with two samples in each test. For tests involving daptomycin, 50 µg mL −1 CaCl 2 is supplemented to the medium. MTT cytotoxicity test Mouse fibroblasts (3T3 cells) were purchased from ATCC. Cells were seeded at 2 × 10 4 cells per well in a volume of 200 μL of Dulbecco’s Modified Eagle’s medium (DMEM, Gibco TM ) in a 96-well tissue culture plate, and incubated at 37 °C in a humidified incubator with 5% CO 2 for 24 h. Polymer stock solution was prepared in PBS (phosphate-buffered saline, Gibco TM ) at a concentration of 10 mg mL −1 and diluted to desired concentrations in DMEM complete medium. Polymer in DMEM solution was added into the cell-seeded 96-well plate and incubated at 37 °C for 24 h. Subsequently cells were rinsed with PBS and 1 mg mL −1 MTT in DMEM was added into each well. The plate was incubated for 4 h, after which the MTT solution was aspirated and 100 μL of dimethyl sulfoxide was added into each well. The plate was shaken at 150 rpm for 10 min and the absorbance of each well was measured at 570 nm using a microplate reader spectrophotometer (BIO-RAD, Benchmark Plus). Cell viability was calculated using the following formula and IC 50 was interpolated using mean values of triplicate measurements. % Cell viability = Average abs of treated cells/Average abs of controls× 100%. (1) Hemolysis assay The human blood hemolysis experiment was reviewed and approved by the Institutional Review Board of Nanyang Technological University (IRB-2015-03-040). Human blood samples were obtained from a healthy donor (age 23, male) and informed consent was given in accordance with NTU-IRB ethical principles. Fresh human blood was washed with PBS twice and red blood cells were resuspended to 5% v/v in PBS. Polymers were twofold serial diluted in PBS and 50 µL of polymer solution samples were mixed with red blood cell suspension in a 96-well plate. The plate was incubated for 1 h at 37 °C under mild shaking. The microplate was centrifuged at 1000 rpm for 10 min; 80-µL aliquots of the supernatant were then transferred to a new 96-well microplate and diluted with another 80 µL of PBS. Hemolytic activity was calculated from absorbance measured at 540 nm using a microplate reader spectrophotometer (Benchmark Plus, BIO-RAD): 
    Hemolysis % = O_p - O_b/O_t - O_b× 100%,
 (2) where O p is the absorbance of polymer, O b is the absorbance of negative control, and O t is the absorbance of positive control. HC 10 values (concentration that causes 10% hemolysis) were interpolated using mean values of triplicate measurements. Kill kinetics of non-replicating/antibiotic-generated persisters A culture of MRSA USA300 was washed two times with PBS and resuspended in PBS at a final concentration of 10 8 CFU mL −1 . The bacteria suspension was incubated in PBS for 1 h to adapt the cells to starvation. Polymer and antibiotic were added to 1 mL of bacteria in PBS suspension in Eppendorf tubes to achieve a desired final polymer/antibiotic concentration. The Eppendorf tubes were incubated aerobically under shaking at 37 °C. At desired time points, 20 µL of each sample was serial diluted in PBS, and plated on nutrient agar plates for CFU determination. For killing of persister bacteria that escaped standard antibiotic treatment, 10 8 CFU log-phase bacteria in 1 mL of MHB were challenged with antibiotics (ciprofloxacin or gentamicin) at 10× MIC for 18 h. Half of the bacteria were washed to remove antibiotics and challenged with copolymer at 4× MIC in MHB. The other half continued under challenge with antibiotics as a control. Aliquots of samples at each time point were washed with PBS twice to remove antibiotics/polymers and serial diluted in PBS to determine CFU. Error bars were produced from two independent tests, with duplicate samples for each test. Spontaneous mutation frequency At day 1, initial inocula of 3.5 × 10 9 CFU exponential-phase MRSA USA300 in 10 mL of MHB were placed in 50-mL falcon tubes and challenged with polymer at 10× MIC under shaking at 37 °C. Polymer was changed every 48 h during the incubation. The OD 600nm values were recorded daily over 6 days. At days 3 and 6, 100 μL of the sample was serially diluted in PBS and plated on nutrient agar plates for CFU determination. Resistance evolution by serial passage Exponential-phase MRSA USA300 (10 6 CFU) were grown in 1 mL of MHB containing copolymer or antibiotic control ciprofloxacin at a gradient of concentrations: 0.25× MIC, 0.5× MIC, 1× MIC, 2× MIC, and 4× MIC. At 24-h intervals, the cultures were checked for growth and the MIC value for each day was recorded. Cultures from the second highest concentrations that allowed growth (OD 600 ≥ 1) were diluted 1:1000 into fresh MHB containing 0.25× MIC, 0.5× MIC, 1× MIC, 2× MIC, and 4× MIC of copolymer/ciprofloxacin. The serial passaging was repeated daily for 14 days. Three independent biological replicates were conducted for each experiment. Microscopic studies Log-phase MRSA USA300 bacteria were washed and diluted to 10 8 CFU mL −1 in PBS and incubated with polymer at 37 °C for 4 h. The bacteria suspension was centrifuged and resuspended in PBS for cryo-TEM imaging. For confocal imaging, 10 8 CFU mL −1 log-phase bacteria were incubated with rhodamine-labeled polymer for 1 h and subsequently stained with membrane dye FM1-43FX before confocal microscopy imaging. Bacterial membrane integrity assays Log-phase bacteria (MRSA USA300) were washed and diluted to 10 8 CFU mL −1 in PBS and incubated with polymer at 37 °C for 0.5 or 1.5 h, and stained with PI (L13152 Invitrogen). Samples were washed twice and resuspended in PBS to 10 7 CFU mL −1 and analyzed using flow cytometry (BD Accuri C6 plus). Data are plotted as normalized histogram of fluorescence intensity from FL3 channel. For DiSC 3 5 membrane depolarization assay, log-phase bacteria were washed and resuspended to 10 7 CFU mL −1 in 5 mM HEPES buffer (pH 7.8) containing 20 mM glucose and 0.1 M KCl. DiSC 3 5 solution was added to bacteria suspension to achieve a final concentration of 100 nM and allowed to quench for 30 min. Polymer solution was added to achieve the desired concentration in a black 96-well plate (Costar). Fluorescence readings were recorded 5 min after polymer addition with a Tecan reader at an excitation wavelength of 622 nm and an emission wavelength of 670 nm. Biofilm assays A total of 150 µL of MRSA USA300 bacteria in tryptic soy broth (TSB) containing 1% glucose (initial inoculum of 10 6 CFU per well) was added into each well of an MBEC plate (Innovotech, Canada). After 24 h of incubation at 37 °C under mild shaking, the pegs were washed twice using 200 µL of PBS and transferred to a 96-well plate containing a twofold dilution series of polymer in PBS (200 µL per well). MBEC pegs were exposed to the polymer for 3.5 h, and subsequently washed before sonication-releasing the biofilm bacteria into the recovery plate for CFU counting. For FESEM imaging of pegs, untreated control and copolymer-treated (64 µg mL −1 for 3.5 h) pegs were removed aseptically, fixed with 4% paraformaldehyde at 4 °C overnight, and dehydrated using a graded ethanol series. For confocal imaging, 24-h preformed biofilm was established in a collagen-coated glass-bottom Petri dish (MatTek). Biofilm was stained with Bac Light™ live/dead kit. Polymer in PBS solution (32 µg mL −1 ) was dropwise added to avoid physical disturbances to biofilm and confocal images were taken immediately after polymer addition and at defined times thereafter. For biofilms formed with polysaccharide intercellular adhesin, various strains of HA-MRSA and MRSE biofilms were established under high-salt conditions using TSB + 4% NaCl. Secondary structure study Polymers were dissolved at 0.05 mg mL −1 in different media, i.e. DI water, 10 mM phosphate buffer (pH 2.6–8.7), 20 mM carbonate buffer (pH 10.8) and in the presence of 1 mg mL −1 POPG or POPC liposomes. (For the POPG liposomes, the polymer:lipid (P:L) molar ratios of PBLK(20) , PDGu(20) , and PDGu(7)- b -PBLK(13) are 1:79, 1:83, and 1:89, respectively.) CD spectra were measured from 190 to 260 nm with 0.5-nm step size, with each measurement performed twice. The final data are presented as the mean values after background extraction. Mouse model of MRSA USA300 infection and in vivo toxicity The animal experiments were reviewed and approved by the Animal Ethics and Welfare Committee (AEWC) of Ningbo University. A single 5-mm-diameter excision wound was created on female C57BL6 mice and inoculated with 2.5 µL of MRSA USA300 suspended in PBS (5 × 10 5 CFU mL −1 ). For treatment initiated at 72 h post-infection, treatments were applied in total six times over 2 days, i.e. three times per day with 4 h between each treatment. Samples were harvested 4 h after the last treatment to determine the CFU. For systemic infection, 10 8 CFU mL −1 MRSA USA300 in PBS (with 5% mucin) were i.p. injected into female balb/c mice and the infections were allowed to develop for 2 h. At 2 h post infection, treatment was injected i.p. at 5 mg kg −1 in 200 μL of PBS. Twenty-four hours post infection, the mice were sacrificed and i.p. fluid, liver, kidney, and spleen were harvested and homogenized to determine the CFU. For survival test, mice were monitored up to 96 h post infection/treatment. For deep-seated thigh infection, neutropenic ICR mice were infected by injecting 50 μL of stationary-phase MRSA USA300 in PBS (10 5 CFU per thigh) into thigh muscles and infection was developed for 24 h. Mice were treated with 20 mg kg −1 copolymer or antibiotic subcutaneously; 3 h later, a second treatment was given by the same route. Thigh tissues were harvested 24 h post first treatment and homogenized to determine the CFU. For in vivo toxicity determination, 10 mg kg −1 of the block copolymer in 200 μL of PBS was injected into female balb/c via tail vein daily for 7 days. 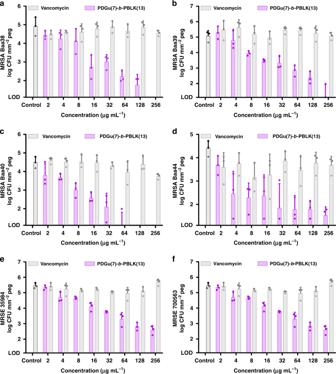Fig. 5 PDGu(7)-b-PBLK(13)eradicates biofilms of HA-MRSA and MRSE strains. It shows dose-dependent eradication of biofilm bacteria under conditions that promote polysaccharide intercellular adhesion;y-axis: biofilm bacteria (CFU mm−2peg) formed by different HA-MRSA strains (aATCC BAA38,bATCC BAA39,cATCC BAA40,dATCC BAA44) and MRSE strains (eATCC 35984,fATCC 700563). (Vancomycin is used as antibiotic control.) Data are presented as mean ± standard deviation 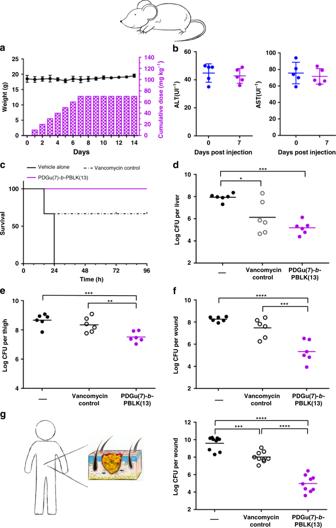Fig. 6 PDGu(7)-b-PBLK(13)is efficacious in vivo against MRSA USA300 with no toxicity.a,bIn vivo repetitive toxicity of daily 10 mg kg−1i.v. injection ofPDGu(7)-b-PBLK(13)for 7 consecutive days.aMice weight (lefty-axis) and cumulative dosage (righty-axis) over 14 days.bALT and AST biomarker changes att= 0 and 7 days. Data are presented as mean ± standard deviation.cSurvival% anddbacteria log reduction in liver in a systemic infection model. Vehicle alone (–),PDGu(7)-b-PBLK(13), or vancomycin control at 5 mg kg−1were applied at a single dose, 2-h post infection.eIn vivo antimicrobial activity ofPDGu(7)-b-PBLK(13)against MRSA USA300 in a deep-seated neutropenic thigh infection model. First treatment was applied 24-h post infection at 20 mg kg−1, with a second dose at 20 mg kg−1applied 3 h later.fIn vivo antimicrobial activity ofPDGu(7)-b-PBLK(13)against MRSA USA300 in an established murine excision wound model. Vehicle alone (–),PDGu(7)-b-PBLK(13), or vancomycin control at the same dosing (i.e. 2.5 mg kg−1) were applied six times over 2 days, starting 72-h post infection.gEx vivo antimicrobial activity ofPDGu(7)-b-PBLK(13)against MRSA USA300 in an established wounded human skin model. Vehicle alone (–),PDGu(7)-b-PBLK(13), or vancomycin control at 100 µg were applied three times with 3-h interval between treatments, starting 48 h post infection; **p≤ 0.01, ***p≤ 0.001, ****p≤ 0.0001 by one-way ANOVA followed by Dunnett test Clinical biomarkers were recorded before, 24 h after, 3 days after, and 7 days after the first injection. For histological analysis, mice were sacrificed at 48 h post final injection and tissues were harvested for H&E staining and examination. Ex vivo wounded human skin infection model Human skin samples were purchased from Biopredic International. All samples were obtained from healthy donors undergoing cosmetic surgery and informed consent was given in accordance with French law and ethical principles. Five-millimeter-diameter wounds were created and inoculated with 10 µL of MRSA USA300 (2 × 10 9 CFU mL −1 ). Infections were developed for 48 h and wound sites were gently rinsed with PBS to remove planktonic bacteria; PBS vehicle alone, 100 µg of vancomycin, or copolymer were applied three times with a 3-h interval between each treatment. Three hours post last treatment, the samples were harvested and homogenized for CFU determination. Reporting summary Further information on research design is available in the Nature Research Reporting Summary linked to this article.